Asymmetric selection and the evolution of extraordinary defences Evolutionary biologists typically predict future evolutionary responses to natural selection by analysing evolution on an adaptive landscape. Much theory assumes symmetric fitness surfaces even though many stabilizing selection gradients deviate from symmetry. Here we revisit Lande’s adaptive landscape and introduce novel analytical theory that includes asymmetric selection. Asymmetric selection and the resulting skewed trait distributions bias equilibrium mean phenotypes away from fitness peaks, usually toward the flatter shoulder of the individual fitness surface. We apply this theory to explain a longstanding paradox in biology and medicine: the evolution of excessive defences against enemies. These so-called extraordinary defences can evolve in response to asymmetrical selection when marginal risks of insufficient defence exceed marginal costs of excessive defence. Eco-evolutionary feedbacks between population abundances and asymmetric selection further exaggerate these defences. Recognizing the effect of asymmetrical selection on evolutionary trajectories will improve the accuracy of predictions and suggest novel explanations for apparent sub-optimality. A fundamental goal in biology is to predict the evolution and optimization of traits in populations undergoing natural selection. Quantitative genetics has emerged as the dominant paradigm for predicting the evolutionary optima for continuous traits [1] . Quantitative genetics has been used to predict the evolution of domesticated crops and animals, natural populations and humans, and thus represents one of the most important tools in modern biology. Lande’s [2] , [3] analytical approach is commonly used to describe the evolution of the mean phenotype on an adaptive landscape [4] . Lande showed that an evolving population climbs the adaptive landscape to a local fitness peak through evolution. In particular, he demonstrated that his equation for the evolution of the mean phenotype can be interpreted as the breeder’s equation used in quantitative genetics. An often-overlooked point (but see refs 5 , 6 , 7 ) is that the adaptive landscape, which assigns the mean fitness of the population to the mean phenotype, can differ from the individual fitness surface, which relates individual fitness to individual trait values. In general, the peaks of the individual fitness surface coincide with the peaks of the adaptive landscape if the population is monomorphic or if both the fitness surface and phenotypic distribution are symmetric and unimodal. Although Gaussian fitness surfaces are often assumed for mathematical convenience, evolutionary biologists have long noted that asymmetric selection is ubiquitous in nature [8] . Here we evaluate the consequences of asymmetrical selection for trait evolution and optimization. A trait determined by many loci should follow a Gaussian distribution owing to the central limit theorem, and indeed normally or log-normally distributed traits are common [9] . In contrast, natural selection need not conform to a Gaussian distribution because it arises from a combination of selection functions rather than the sum of random variables as for quantitative traits. Individual fitness surfaces so frequently diverge from the Gaussian distribution [10] that more flexible statistical fitting methods such as the cubic spline are usually employed to characterize fitness surfaces [8] . If natural selection is frequently asymmetric, then how does this affect the evolution of quantitative traits? Parker and Smith [11] presented a verbal argument that an asymmetric fitness surface would bias the equilibrium mean phenotype away from the individual fitness optimum. This possibility has been used to explain apparently suboptimal mean clutch sizes in birds and body sizes in Drosophila [12] , [13] . However, no general theory has been derived to predict the direction or extent of this bias for an asymmetric fitness surface. Here we develop analytical theory and genetic simulations that incorporate skewed phenotypic distributions to predict the effects of asymmetric fitness surfaces on evolutionary equilibria. We then apply this theory to explain an apparent paradox in biology: why do excessive and costly defensive traits sometimes evolve contrary to what is expected based on individual fitness? We show that asymmetric selection can strongly bias evolutionary responses and that this asymmetric selection can produce extraordinary defences and thereby explain autoimmune responses and other excessive investments in defence. Evidence for asymmetric selection Although examples of symmetric stabilizing selection exist (for example, Bumpus’ sparrows, Fig. 1a ), many individual fitness distributions are skewed ( Fig. 1b–d ). Examples of asymmetric selection include human birth weight [14] ( Fig. 1b ), parasitic gall size [15] ( Fig. 1c ), and bill depth in Darwin’s finches ( Geospiza spp.) [16] . In this last example, stabilizing selection on bill depth is strongly left-skewed, having a flatter shoulder for smaller-than-optimal bill depths ( Fig. 1d ) [16] . Other traits subject to asymmetric selection but not displayed include bird clutch size [12] and insect body size [13] . 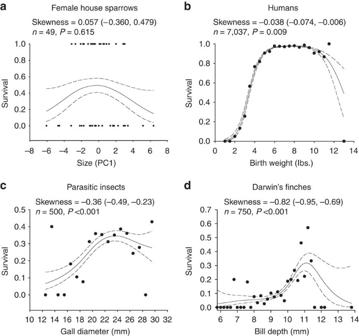Figure 1: Iconic examples of stabilizing selection. Examples are arranged in order of increasingly negative skewness, where the left tail is flatter, including (a) survival of house sparrows based on body size32, (b) human baby survival based on birth weight14, (c) survival of the parasitic insectEurosta solidaginisfrom 1984–1985 based on gall diameter15and (d) survival of Darwin’s finches (Geospizaspp.) on Daphne Island from 1976–1978 (including immigrant birds) based on bill depth16. Lines indicate the best cubic spline fit (±1 s.e.m.) as per Schluter8. For presentation, we bin survival data in large datasets and depict average survival. To calculate skewness, we first estimated predicted values for 200 equally spaced points across the range of trait values to discretize the smoothed fitness surface to avoid giving undue weight to outliers. We then calculated 10,000 estimates of skewness using the original number of samples with replacement and with probability equal to relative fitness. We calculated 95% confidence intervals around mean skewness and the probability that skewness was zero or opposite in sign from estimated mean skewness. Figure 1: Iconic examples of stabilizing selection. Examples are arranged in order of increasingly negative skewness, where the left tail is flatter, including ( a ) survival of house sparrows based on body size [32] , ( b ) human baby survival based on birth weight [14] , ( c ) survival of the parasitic insect Eurosta solidaginis from 1984–1985 based on gall diameter [15] and ( d ) survival of Darwin’s finches ( Geospiza spp.) on Daphne Island from 1976–1978 (including immigrant birds) based on bill depth [16] . Lines indicate the best cubic spline fit (±1 s.e.m.) as per Schluter [8] . For presentation, we bin survival data in large datasets and depict average survival. To calculate skewness, we first estimated predicted values for 200 equally spaced points across the range of trait values to discretize the smoothed fitness surface to avoid giving undue weight to outliers. We then calculated 10,000 estimates of skewness using the original number of samples with replacement and with probability equal to relative fitness. We calculated 95% confidence intervals around mean skewness and the probability that skewness was zero or opposite in sign from estimated mean skewness. Full size image Evolution under asymmetric selection Here, we show how asymmetric selection shifts the mode of the adaptive landscape, that is, the mean fitness function , toward the flatter shoulder of the individual fitness surface. We provide general conditions for the direction of this shift and demonstrate this principle by modelling trait evolution using two qualitatively different skewed individual fitness surfaces. First, we approximate the slopes of the fitness surface with a cubic polynomial function in equation (3) and then find the condition when the optimum of mean fitness is shifted to the right of the optimum of the individual fitness surface (equation (4), and Supplementary Methods , Supplementary equations (S1–S4) ). Then we modify the classical Gaussian fitness surface by multiplying it by a linear function and renormalizing it in equation (5), which closely approximates the skew-normal distribution ( Fig. 2a ) [17] . The shape parameter ψ determines the degree and direction of skew. Negative ψ generates left skew, positive ψ generates right skew and the Gaussian distribution is recovered when ψ =0. By applying our polynomial method to the skew-normal distribution, we can show that equation (4) is always satisfied and the optimum of mean fitness is shifted to the right (equation (6)). In a later section, we evaluate a skewed individual fitness function based on assumptions about selection from enemies on victim traits. 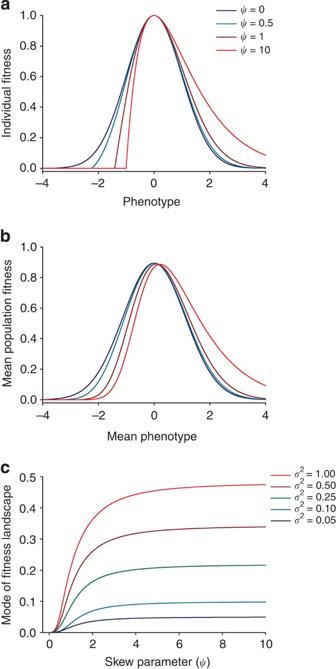Figure 2:Skew affects individual fitness surfaces and adaptive landscapes. (a) The individual fitness surface becomes more skewed with increasingψ, ranging from a symmetric Gaussian distribution (dark blue) to a highly skewed distribution (red). We fix the mode of individual fitness surface at zero and strength (curvature) of stabilizing selection at −1 (equation (5)). (b) The mean population fitness depending on mean population phenotype (that is, the adaptive landscape) based on the same individual fitness curves in (a) and assumingσ2=0.25. (c) The mode of the adaptive landscape diverges from the optimum of the individual fitness surface in (a), which is set to zero with increasing skew andσ. Figure 2: Skew affects individual fitness surfaces and adaptive landscapes . ( a ) The individual fitness surface becomes more skewed with increasing ψ , ranging from a symmetric Gaussian distribution (dark blue) to a highly skewed distribution (red). We fix the mode of individual fitness surface at zero and strength (curvature) of stabilizing selection at −1 (equation (5)). ( b ) The mean population fitness depending on mean population phenotype (that is, the adaptive landscape) based on the same individual fitness curves in ( a ) and assuming σ 2 =0.25. ( c ) The mode of the adaptive landscape diverges from the optimum of the individual fitness surface in ( a ), which is set to zero with increasing skew and σ . Full size image In general, the adaptive landscape is calculated as the integral of the individual fitness surface multiplied by the density of the trait distribution. In Methods and Supplementary Methods , we obtain explicit analytical results. We show that increasingly asymmetrical selection shifts the optimum mean phenotype (the mode of the adaptive landscape) toward the flatter shoulder of the individual fitness surface which, for our skew-normal distribution, is also toward the longer tail: right for positive skew and left for negative skew ( Fig. 2b ). The magnitude of this shift increases with higher skew in the fitness surface and with higher phenotypic variance ( Fig. 2c ). Intuitively, this bias arises because when a population’s mean phenotype is at the peak of an asymmetric fitness surface, individuals on the flatter shoulder of the individual fitness surface will be more fit than individuals on the steeper shoulder. Consequently, directional selection can still change the trait mean even when it is at the peak. Asymmetric selection also indirectly affects the equilibrium mean phenotype, because it changes the shape of the trait distribution which, in turn, modifies the response to selection. Lande’s theory for the response of the mean of normally distributed traits can be generalized [18] , [19] to account for this effect. For non-Gaussian distributions of breeding values, the mean response can be written as where is the genetic variance, C k denotes the k th cumulant of the distribution of breeding values, L k = is the selection gradient of order k , and M is the contribution from asymmetric mutation [20] . If we ignore terms involving cumulants of order higher than three, the following condition is met at equilibrium ( ). where L 1 and L 2 are the directional and stabilizing selection gradients, respectively, of the distribution of breeding values. If M is sufficiently small, the sign of directional selection ( L 1 ) will match that of skewness ( C 3 ), because stabilizing selection always induces negative L 2 and genetic variance ( σ 2 ) is always positive. For positive skew, the mean phenotype will equilibrate where directional selection is positive, that is, to the left of the optimum of the adaptive landscape (but not necessarily the individual fitness surface) and to the right when skew is negative. Hence, asymmetric natural selection has two opposing effects on evolution: it directly biases the equilibrium mean trait toward the flatter shoulder of the individual fitness surface and indirectly biases it toward the steeper shoulder via effects from a skewed phenotypic distribution. The cumulative effect of these opposing forces depends both on the kind of asymmetry of the individual fitness surface and the population’s phenotypic variance (See Supplementary Fig. S1 ). The selection differentials L 1 and L 2 can be calculated as functions of ψ , σ 2 and for the skew-normal distribution (see Supplementary Methods , Supplementary equations (S5–S10) ). Except for special cases reviewed in Bürger [20] , no theory is available to calculate the equilibrium values of , σ 2 and C 3 , because they depend on the specific genetic details [18] , [19] , [20] , [21] . Nevertheless, they can be determined from genetic simulations and entered into equation (2) to predict from σ 2 and C 3 . Equation (1) for the evolutionary response of the mean holds quite generally for randomly mating sexual populations with equivalent sexes or for asexually reproducing populations provided the trait is determined additively by a finite number of loci. It holds independently of the population size, of the number and effects of loci, and of linkage relations. The response of the variance and the higher cumulants is much more complicated and depends on genetic details, even if linkage disequilibria are weak or absent [18] , [19] , [20] , [21] , [22] . Although selection will cause deviations from a normal distribution of breeding and phenotypic values directly and indirectly via linkage disequilibria, such deviations do not change the central relations in equations (1) or (2),; they do influence, however, the cumulants and selection gradients. In addition, as shown in Supplementary Methods ( Supplementary equations (S11–S13) ), the first-order and second-order selection gradients ( L 1 and L 2 ) are, to leading order, independent of the skew or higher cumulants of the distribution of breeding values. Therefore, our results agree with Turelli and Barton [21] that the assumption of a normal distribution of breeding values in calculating the selection response gives remarkably accurate predictions for the mean and variance. In accordance with theoretical predictions, our genetic simulations show that asymmetric selection usually biases the mean phenotype at equilibrium toward the flatter shoulder of the distribution, that is, to the right for positive skew and to the left for negative skew ( Fig. 3 ). Higher ψ -values increase skew in the individual fitness surface, which in turn accentuates the bias in the mean phenotype. It is theoretically possible for effects via the skewed trait distribution to shift optima toward the steeper shoulder (see Supplementary Fig. S1 ). However, in our simulations, we could not find parameters that generate enough phenotypic skew to overcome the direct effect of asymmetric selection which displaces the mean to the right and thereby displace the mean phenotype to the left (steeper shoulder) of the adaptive landscape (equation (2)). Consequently, bias in the direction of the flatter shoulder of an asymmetric fitness surface might be most common. 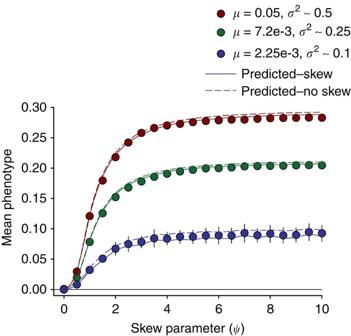Figure 3: Analytical results predict simulated evolution of mean phenotypes. The equilibrium mean phenotype calculated from simulations (n=50; circles ±s.e.m.) becomes increasingly divergent from the individual fitness optimum at zero with higherψ, which increases skewness. The equilibrium mean phenotype also increases with higher mutation rates (μ), which determine genetic variances (σ2). We also plot theoretical predictions with (solid line) and without (broken line) skewness incorporated. Theory that includes the effect of skewness (solid line) predicts genetic simulation results. Parameters not listed in the inset areK=5000,forμ=0.00225 andμ=0.0072, andforμ=0.05. Figure 3: Analytical results predict simulated evolution of mean phenotypes. The equilibrium mean phenotype calculated from simulations ( n =50; circles ±s.e.m.) becomes increasingly divergent from the individual fitness optimum at zero with higher ψ , which increases skewness. The equilibrium mean phenotype also increases with higher mutation rates ( μ ), which determine genetic variances ( σ 2 ). We also plot theoretical predictions with (solid line) and without (broken line) skewness incorporated. Theory that includes the effect of skewness (solid line) predicts genetic simulation results. Parameters not listed in the inset are K =5000, for μ =0.00225 and μ =0.0072, and for μ =0.05. Full size image Increasing phenotypic variance in a population also increases the displacement of equilibrium trait means. A greater phenotypic variance allows for stronger sampling of the higher relative fitness in the flatter shoulder (and long tail) and its integration into population fitness. Comparison of theoretical predictions and simulation results demonstrates that our analytical theory accurately explains the observed deviation in the optimal mean phenotype from the individual fitness optimum ( Fig. 3 ), even though our approximation ignores the influence of deviations of the trait distribution from Gaussian on the adaptive landscape, the influence of cumulants of higher order on selection responses and random genetic drift in the simulated finite populations. Evolution of extraordinary defences We next apply this theory to an apparent paradox in evolutionary biology. A defensive trait generally evolves as a compromise between its efficacy against enemy attacks and the fitness costs associated with developing and maintaining the defence [23] . However, despite costs of defence, sometimes victims evolve defences that far exceed the level that is sufficient to defend against an enemy, hereafter termed ‘extraordinary defences.’ As an example, many organisms, including humans, develop autoimmune disorders, which effectively defend against enemies but compromise fitness by attacking healthy tissue [24] , [25] . As a consequence, some individuals in a population might be vulnerable to anaphylactic shock, in which comparatively harmless allergens provoke potentially fatal systemic immune reactions. In a predator–prey example, snails from freshwater springs in northern Mexico develop shells that are 2–3 times harder than is necessary to withstand the maximum biting force of the local molluscivorous cichlid fish [26] . Such defences have been attributed to environment-dependent fitness costs of defences [26] and historical, but now absent, selection [25] . However, we offer a simple explanation that only requires asymmetric selection and phenotypic variance, both of which are universal properties of natural systems. We develop a model in which a victim population can evolve defences against the enemy population (see Methods and Supplementary Methods for details). We create an asymmetric individual fitness surface such that fitness is skewed toward greater predator defence. We expect this fitness asymmetry to be quite general, because insufficient defence often will be fatal whereas excessive defence might only incur more trivial energetic costs. We assume that victim survival is positively and exponentially related to defence up to a threshold in equation (7). Beyond this threshold, the victim becomes invulnerable ( Fig. 4a ). For example, shell thickness, body size or an immune response can provide increasing protection against enemies up to a level at which the victim becomes invulnerable [27] . We assume that fecundity declines linearly with increasing investment in defences because energy allocated to defence would otherwise be allocated to reproduction [28] . This decline becomes most evident in the model when victims have defence levels exceeding the invulnerability threshold (left side in Fig. 4a ) where defence benefits no longer counter fitness costs. We assume a predator population with discrete population dynamics where birth rate is proportional to prey consumed and assuming a fixed death rate in equation (8). 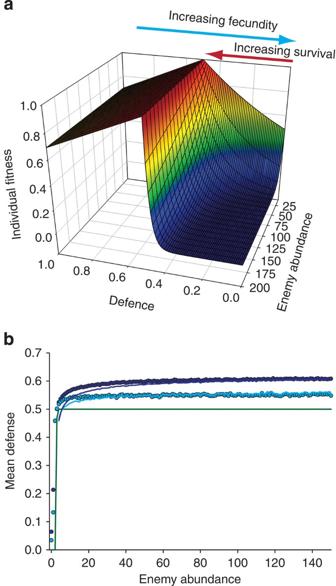Figure 4: Asymmetric selection causes evolution of extraordinary defences. Fitness surfaces and mean defences differ based on enemy abundance and intraspecific variance. (a) Survival increases from right to left up to a point of invulnerability when defence levels=0.5 (red arrow; equation 7). Fecundity increases toward the right because we assume that investment in defence has a fecundity cost (blue arrow). This fecundity cost is most visible beyond the point of invulnerability. From back to front, enemy abundance increases. Increased enemy abundance increases the asymmetrical selection for defences even though the peak of the individual fitness surface remains constant at 0.5. Parameters:amax=0.1,γ=0.2,c=0.6,N=10,K=2,000,. (b) The mean equilibrium defence differs depending on enemy abundance and trait variance in the victim population. Without intraspecific variance, the optimal defence equals 0.5 when predator density >4 (green line). With intraspecific variance, the optimal defence exceeds 0.5 for most enemy densities (blue symbols) with greater divergence when variance is higher (light blue symbols,σ2≈0.0015; dark blue symbols,σ2≈0.0035). Theoretical predictions (solid lines) predict mean defence optima (n=50) ±3%. Same parameters used as for (a) exceptNis dynamic andμ=1e-3 and 5e-4 for the low and high variance simulations, respectively, andb=0.05,d=0.02. Figure 4: Asymmetric selection causes evolution of extraordinary defences. Fitness surfaces and mean defences differ based on enemy abundance and intraspecific variance. ( a ) Survival increases from right to left up to a point of invulnerability when defence levels=0.5 (red arrow; equation 7). Fecundity increases toward the right because we assume that investment in defence has a fecundity cost (blue arrow). This fecundity cost is most visible beyond the point of invulnerability. From back to front, enemy abundance increases. Increased enemy abundance increases the asymmetrical selection for defences even though the peak of the individual fitness surface remains constant at 0.5. Parameters: a max =0.1, γ =0.2, c =0.6, N =10, K =2,000, . ( b ) The mean equilibrium defence differs depending on enemy abundance and trait variance in the victim population. Without intraspecific variance, the optimal defence equals 0.5 when predator density >4 (green line). With intraspecific variance, the optimal defence exceeds 0.5 for most enemy densities (blue symbols) with greater divergence when variance is higher (light blue symbols, σ 2 ≈0.0015; dark blue symbols, σ 2 ≈0.0035). Theoretical predictions (solid lines) predict mean defence optima ( n =50) ±3%. Same parameters used as for ( a ) except N is dynamic and μ =1e-3 and 5e-4 for the low and high variance simulations, respectively, and b =0.05, d =0.02. Full size image The mean fitness of the population reaches a maximum when the population is just invulnerable but does not invest any more into costly defences (optimal defence=0.5; Fig. 4b ; green line). However, with intraspecific trait variance, we observe a displacement in equilibrium defence values toward the flatter shoulder of the individual fitness surface as predicted by our analytical theory. This bias increases with increasing trait variance ( Fig. 4b , compare dark blue versus light blue symbols). The approximate theoretical predictions match simulation results well when enemy abundances are large ( Fig. 4b , theoretical predictions as lines) despite ignoring higher-order terms and other processes. Theory underestimates mean defences at low predator abundances, because fecundity selection overwhelms mortality selection and equation (7) no longer accurately represents the two combined phases of selection. In addition, at very low enemy abundances, the mode of selection occurs outside the phenotypic range and theory no longer applies. Eco-evolutionary feedbacks [29] further amplify the difference between individual optima and the equilibrium trait mean. Phenotypic variation among victims generates maladapted individuals with lower defences than the optimal value. These individuals subsidize enemy reproduction leading to higher enemy abundance than occurs for a homogeneous population with the optimal defence. More enemies generate greater mortality risk for under-defended individuals that, in turn, results in a more asymmetric fitness surface ( Fig. 4b , moving from left to right). This greater asymmetry then increases the optimal investment in defences. In the representative dynamic in Fig. 5 based on simulations of Equations (7) and (8), we display (a) victim and enemy abundances through time and (b) the evolution of prey defences relative to enemy abundances through time. Victims evolve from an initial defence value of 0.5 (which is optimal without asymmetrical selection or trait variation) to 0.59 in 5 generations (dashed vertical line), which is the optimal defence predicted from numerical simulations based on genetic variance and fixed enemy population size ( Fig. 5b ). However, maladapted victims augment the enemy population, maintaining it well above the initial abundance of ten ( Fig. 5a ). A stable eco-evolutionary equilibrium is reached after 120 generations when the enemy population size stabilizes at 100 and victim defences evolve to 0.7. 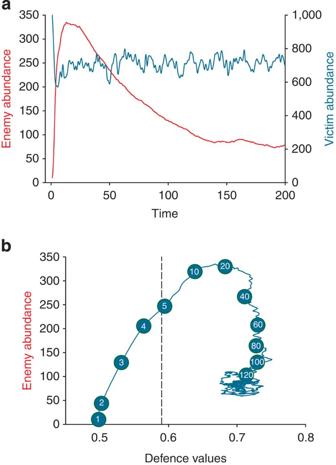Figure 5: Eco-evolutionary dynamics enhance asymmetric selection. In (a), enemy (red) and victim (blue) abundances are shown through time. In (b), enemy abundance is depicted relative to mean victim defences (generation number is shown in numbered circles). The dashed line indicates the optimal defence without intraspecific variance given the initial predator abundance. Parameters are the same as forFig. 4bhigh variance simulations exceptc=0.2. Figure 5: Eco-evolutionary dynamics enhance asymmetric selection. In ( a ), enemy (red) and victim (blue) abundances are shown through time. In ( b ), enemy abundance is depicted relative to mean victim defences (generation number is shown in numbered circles). The dashed line indicates the optimal defence without intraspecific variance given the initial predator abundance. Parameters are the same as for Fig. 4b high variance simulations except c =0.2. Full size image Quantitative genetics is the primary tool for predicting the evolutionary responses of continuous traits to natural selection. For mathematical convenience, mostly symmetrical fitness surfaces have been assumed when studying evolution of quantitative traits under stabilizing selection. Yet, fitness surfaces often are not symmetrical. For instance, evolutionary biologists frequently use cubic splines to represent non-Gaussian surfaces [8] . On non-Gaussian fitness surfaces, a population’s equilibrium trait mean need not match the peak of the individual fitness surface. Previous research has explored the divergence between the adaptive landscape and individual fitness surfaces that are bimodal [6] and in a ridge and saddle configuration [7] . Here we explore the general case of asymmetrical selection, which is commonly encountered in nature ( Fig. 1 ). Our theory predicts that evolutionary outcomes can diverge strongly from the peak of the individual fitness surface when asymmetry is pronounced and populations vary phenotypically. This theory incorporates both the direct effects of asymmetric selection on the optimum mean phenotype and the indirect effects via skew in the distribution of breeding values. Asymmetric selection and phenotypic variance are likely to be ubiquitous in nature, and thus we expect this deviation in evolutionary optima from the peak of the individual fitness surface to be quite common. Existing theory will suffice for selection that is relatively symmetrical. However, when faced with strong asymmetry in selection, practitioners of quantitative genetics must consider the skewness—not just the mean and variance—of fitness surfaces as is commonly practiced. An asymmetric fitness surface directly shifts the optimum mean phenotype toward its flatter shoulder. In this part of the fitness surface, the marginal cost of deviating from the optimum is small compared with the marginal cost of deviations on the other side [10] , [13] . Greater variance amplifies this evolutionary bias by ensuring greater sampling of asymmetrical fitness outcomes ( Fig. 2c ), a result also shown numerically for Drosophila body size [13] . The indirect effect of asymmetric selection occurs because a skewed genotypic distribution also modifies the selection response. This biases the mean phenotype toward the steeper shoulder, thus opposing the direct effect. Genetic simulations suggest that the direct effect usually dominates, and populations generally evolve a mean trait shifted toward the flatter shoulder of the fitness surface. However, opposite effects are theoretically possible with strong trait skew and high population variance or with environmental variance that further skews phenotypic distributions (for example, Yoshimura et al. [30] ). We also show that considering asymmetrical selection can be vital to understanding the evolutionary optima of ecologically important traits. We evaluate how asymmetrical selection affects the evolutionary dynamics of enemy defences. We assumed two simple functions for fitness: (1) a linear decline in fecundity due to costs of higher defence and (2) an exponential increase in predation risk with lower defence. Together, these fitness functions create an individual fitness surface that is skewed toward greater defence ( Fig. 4a ). Simulations confirm that effects of skew on the evolution of defence can be substantial. Our example shows that greater skew and higher population variance increase mean investment in the trait up to a 22% more than predicted based on individual fitness alone ( Fig. 4b ), with higher biases possible if we assumed higher phenotypic variance or more strongly skewed selection surfaces. Results highlight the importance of phenotypic variance in altering both evolutionary and ecological dynamics [31] . Moreover, eco-evolutionary dynamics amplify these effects because maladapted victim populations promote larger enemy populations, thereby increasing selection skew and subsequent evolutionary bias ( Fig. 5 ). As less defended victims are likely to enhance enemy populations, such eco-evolutionary amplification might be a common way that extraordinary defences emerge from natural species interactions. Through both shifts in optima and eco-evolutionary amplification, asymmetric selection provides a general explanation for the apparent over-investment in defences. Asymmetric selection could provide a general explanation for the evolution of autoimmune diseases, such as type-I diabetes, rheumatoid arthritis and multiple sclerosis; these debilitating disorders affect a subset of individuals within a population as a side effect of strong average immune function. Similarly, asymmetric selection might explain excessive levels of costly anti-predator defences [26] . Often, the per capita mortality costs of low defence are likely to exceed the per capita fitness costs of investment in predator defences. As a result, it might not be necessary to invoke more complicated scenarios in which excessive defences result from the residual effect of stronger selection in the past. Although we highlight how asymmetrical selection alters defence optima here, such selection will alter the evolution of any quantitative trait regardless of function (for example, see Mountford [12] and Yoshimura et al. [13] ). Future empirical work will be needed to test this theory. In most cases, biologists have not explored asymmetric stabilizing selection as an explanation simply because as a discipline we have usually assumed symmetry. We predict that a greater appreciation of asymmetrical selection and its effects on evolution will improve the accuracy of evolutionary predictions and explain additional paradoxes in phenotypic evolution. Asymmetric stabilizing selection and the adaptive landscape We assume an asymmetric individual fitness surface. Unless the phenotypic variance is unusually large, it is sufficient to describe the fitness surface near its optimum. We approximate the two slopes of the fitness surface by polynomials of degree three. Essentially, we describe the individual fitness surface by its first three derivatives to the left and right of the optimum. More precisely, we assume If we require that the individual optimum is at x =0 (and w (0)=1), we must have a 1 ≤0 and b 1 ≥0. The first line in equation (3) describes the shape of the right shoulder, and the second that of the left shoulder. A Gaussian or quadratic function with optimum at 0 satisfies a 1 = b 1 = a 3 = b 3 =0 and a 2 = b 2 =− s , where s >0 measures the strength of stabilizing selection. More generally, a fitness surface that is smooth and describes stabilizing selection with optimum at 0 satisfies a 1 = b 1 =0 and a 2 = b 2 <0. Symmetric fitness functions satisfy a 1 =− b 1 ≤0, a 2 = b 2 ≤0 and a 3 =− b 3 . We calculate the mean fitness given a Gaussian phenotype distribution in Supplementary Methods , Supplementary equation (S1) . If σ 2 denotes the phenotypic variance, we find the following condition for the optimum of mean fitness to be positive, that is, shifted to the right of the optimum of the individual fitness surface: In general, this implies that the optimum of mean fitness is shifted to the flatter shoulder of the individual fitness surface. If the individual fitness surface has derivatives of order one and two, hence a 1 = b 1 =0, a 2 = b 2 <0, then this condition becomes a 3 + b 3 >0. If a 1 + b 1 >0 and a 2 and b 2 do not differ greatly, then the right shoulder is flatter, and the above condition will be satisfied for the majority of the parameter range if σ 2 is small. We model stabilizing selection by a modified skew-normal distribution: where ψ determines skew. This fitness function has its optimum at x =0, where it assumes w (0)=1, a long right tail and steep left shoulder (see Fig. 2 ). The curvature of w ( x ) at the optimum, which describes the strength of stabilizing selection, is −1. If ψ =0, then w ( x ) becomes Gaussian with optimum 0 and curvature −1. Assuming a Gaussian phenotypic distribution, the mean fitness and its mode are given in Supplementary Methods , Supplementary equations (S5) and (S10) . Both higher skew and higher phenotypic variance inflate the distance between the modes of the adaptive landscape and of the individual fitness surface ( Fig. 2c ). We also note that in terms of the fitness function considered in equation (5), we obtain for (3): Therefore, equation (4) is always satisfied and the mode is shifted to positive values. Evolution under asymmetric selection Under asymmetric selection, mean phenotypes evolve according to equation (1) in the main text, and equation (2) provides an approximate condition for equilibrium. From the formula for equilibrium mean fitness (see Supplementary Methods , Supplementary equation (S5)) , we obtain explicit (but approximate) expressions for the selection differentials L 1 and L 2 as functions of ψ , and σ 2 ( Supplementary Methods , Supplementary equations (S6–S9)) . Substituting these expressions into equation (1), we obtain the relationships between , σ 2 , C 3 and ψ that must be approximately satisfied at equilibrium. We determine equilibrium values based on genetic parameters derived from individual-based simulations. In individual-based genetic simulations, we assume N haploid individuals with discrete annual dynamics with a trait determined additively by 20 biallelic loci with equal effects ± δ . Individuals survive with a probability equal to their fitness along the asymmetric fitness surface in equation 5. After viability selection, surviving individuals are paired to become parents through random sampling with replacement until the population reaches carrying capacity K . Offspring have a genotype sampled randomly from both parents with mutations occurring with rate μ . We explored three mutation rates that produced genetic variances of ~0.1, 0.25 and 0.50. We ran 50 simulations for each combination of ψ and μ for 25,000 generations, which ensured that the population reached quasi-equilibrium. Estimated σ 2 and C 3 from simulations were substituted into equation (2) to calculate the expected equilibrium mean phenotype, . As there is recurrent mutation between the two alleles at each locus, mutation generally influences the between-generation change of the mean and reduces skewness. The change in the mean caused by mutation is (see equations (1) and (2)). For the cases with a high mutation rate, not only does this change the mean but also the skew-reducing effect of mutation is quite large. This is the reason why in Fig. 3 the difference between the predictions ignoring and invoking skew is small. For symmetric mutation models such as the random walk model by Bürger [20] , this difference will be larger. Evolution of extraordinary defences We similarly developed a stochastic individual-based simulation for an evolving victim population with discrete logistic population dynamics, but in response to an asymmetric fitness surface generated by defences against an enemy population. The individual fitness surface can be approximated by when predation-induced mortality is strong relative to fecundity selection. In the genetic simulations, individuals first undergo mortality selection. Victim survival declines exponentially with predator density P times the predator’s maximum attack rate a max minus the decrease in enemy attack with increasing defence γ ( x ). After mortality selection, surviving individuals reproduce sexually. In this step, fecundity declines linearly with a cost to defence investment c . Predator population dynamics were determined by the total number of victims eaten, e , and fixed death birth and death rates: The defensive trait was determined additively by 20 biallelic haploid loci. We randomly mated surviving individuals to produce offspring with clutch size determined as a Poisson realization of the mean fecundity of the two parents. Offspring have a genotype sampled randomly from both parents with mutation rate μ , which we varied to alter population variances. We ran 50 simulations for each parameter evaluated for 10,000 generations, which ensured that the populations reached quasi-equilibrium. A detailed account of the analytical theory is provided in the Supplementary Methods ( Supplementary equations (S14–S16) ). How to cite this article: Urban, M.C. et al. Asymmetric selection and the evolution of extraordinary defences. Nat. Commun. 4:2085 doi: 10.1038/ncomms3085 (2013).